Correspondence: Reply to ‘On the bonding in ligand-protected gold clusters’ 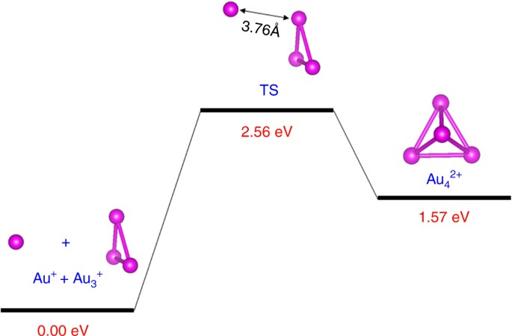Fig. 1 The computed reaction pathway for the Au++ Au3+← → Au42+reaction. Color code: Au—magenta 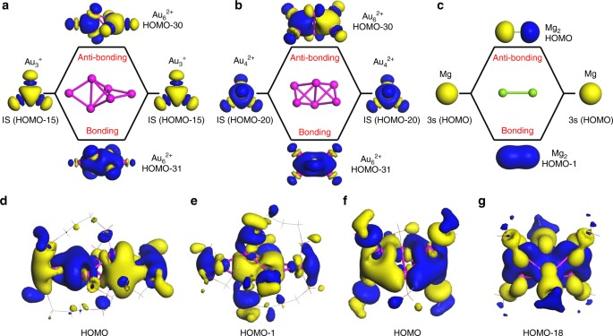Fig. 2 The anti-bonding and bonding orbital diagrams of clusters.aD2dAu62+,bD2hAu62+, andcMg2. The HOMOdand HOMO-1eof [Au6(dppp)4]2+, HOMOf, and HOMO-18gof [Au6(PR3)6]2+. Color code: Au—magenta, Mg—green In the recent Correspondence [1] , Professor Henrik Grönbeck made several comments on the recently developed grand unified model (GUM) [2] , in particular using the ligand-protected gold cluster [Au 25 (SR) 18 ] 1− as an example. We noted that the latter cluster can be viewed as belonging to a special group of ligand-protected gold clusters that contain one or several icosahedral Au 13 motifs [3] . For this group of clusters, a secondary block Au 13 (8 e ) has been identified as a more convenient way to describe their structure anatomy and evolution. Another extension of the GUM is the identification of the new elementary block, Au 3 ( μ 3 -S), with zero valence electron [referred as Au 3 ( μ 3 -S)(0 e )] to describe all crystallized ligand-protected gold clusters containing μ 3 -S motifs [4] . In this correspondence, first, we discuss the purpose of GUM development in more detail. Next, we briefly discuss the secondary block Au 13 (8 e ) and show new computational results on the stabilities of Au 3 (2 e ) and Au 4 (2 e ) elementary blocks. Then two Au 6 2+ clusters are used as the simplest example (a suggestion credited to a reviewer of ref. [2] ) to better explain the GUM and high stability of Au 3 (2 e ), followed by a summary and perspective. Purpose of GUM development : First of all, we reiterate a statement pointed out clearly in the abstract of ref. [2] , that is, “GUM is a predictive heuristic and may not be necessarily reflective of the actual electronic structure”. In other words, the development of GUM is not intended to describe actual electronic structures or electron re-hybridization within the Au core or between the Au core and ligands at atomic level. Density functional theory (DFT) can already serve that purpose. GUM is a model to highlight a universal correlation between the number of valence electrons in the Au core and the number of elementary blocks, with consideration of the ligand effect. As a rule of thumb, GUM can be used to describe structure anatomy and evolution of the ligand-protected clusters. When using the GUM, the focus is placed on treating the ligand-protected clusters in a coarse-grained fashion in terms of elementary blocks [2] or secondary blocks [3] , while the counting of valence electrons is at the elementary block level. As such, the assignments of the 1 valence electron for Au atom in the Au core, 0 valence electron for the PR 3 ligand, and −1 valence electron for halides are empirical descriptions of electronic structure of the ligand-protected gold clusters. Such a description is not intended to reflect the exact electron distribution at the atomic level because these assignments neglect many details in atomic level electronic structures, such as the s – d hybridization, spin-orbit effects, ligands’ constraint effects, etc. Nevertheless, these detailed assignments of valence electrons and valence electron counting are widely used as rules of thumbs in general chemistry and hence employed in GUM as well. In summary, the development of GUM is to introduce a generic rule of thumb—a rule derived after analyzing a “big data” of all 71 clusters available in the literature. In practice, we would like the GUM to be used simply as a rule of thumb, particularly for the design and prediction of new ligand-protected Au clusters. If a new ligand-protected cluster, either designed from theory or determined based on mass spectroscopy or transmission electron microscopy (TEM) experiments, does not satisfy the rule of thumb as described in GUM, the predicted structure of the cluster would be questionable or likely unrealistic for next step crystallization effort. A secondary block icosahedral Au 13 (8e) : Among the 71 ligand-protected clusters illustrated in ref. [2] , there is a special group of ligand-protected gold nanoclusters that all contain one or several icosahedral Au 13 motifs. For these ligand-protected clusters, according to the electron counting protocols for effective detachment of ligands in GUM, each icosahedral Au 13 motif can be assigned to have 8 e valence electrons [Au 13 (8 e )], as each icosahedral Au 13 motif can be viewed as packing of four elementary blocks. For example, the Au 13 (8 e ) in [Au 25 (SR) 18 ] 1− consists of two Au 3 (2 e ) and two Au 4 (2 e ) elementary blocks. Note that this decomposition is not intended to reflect the electronic structure of the Au 13 core at the atomic level but simply to indicate that the 8 e valence electrons of Au 13 (8 e ) can be viewed as a sum of four pairs of valence electrons of the four elementary blocks. Au 13 (8 e ) can be also viewed as an electron shell closure species, in analog of that of the stable Ne atom. As such, the Au 13 (8 e ) may be regarded as a secondary block (or coarse-grained block) to constitute the gold cores of the special group of ligand-protected gold clusters with one or several icosahedral Au 13 motifs. The introduction of secondary block Au 13 (8 e ) into GUM appears to be a convenient supplement to understand this special group of ligand-protected gold clusters with icosahedral Au 13 motifs. It can be also exploited for predicting new ligand-protected gold clusters by design (see ref. [3] for more detail). Stabilities of Au 3 (2e) and Au 4 (2e) : The high stabilities of the trimer Au 3 (2 e ) and tetramer Au 4 (2 e ) elementary blocks are in part due to the strong electronic delocalization among the three- and four-Au atom clusters, and associated strong electron shell closure. From the computed formation energy (Supplementary Table 3 in ref. [2] ), one can see that the Au 4 (2 e ), although not as stable as Au 3 (2 e ), is still highly favorable in formation energy, compared to the isoelectronic dimer Au 2 . In addition, the dissociation barrier from Au 4 2+ to Au 3 + and Au + is computed to be ~1 eV (Fig. 1 ), suggesting the Au 4 2+ can be a stable species in the gas phase at room temperature. Thus, Au 3 + and Au 4 2+ , if could be made in the laboratory, would very likely be a standing-alone/stable species without the ligand protection, largely due to the strong electronic delocalization among Au 3 + and Au 4 2+ , and associated strong electron shell closure. Fig. 1 The computed reaction pathway for the Au + + Au 3 + ← → Au 4 2+ reaction. Color code: Au—magenta Full size image Using Au 6 2+ as the simplest example to illustrate GUM : Here, two Au 6 2+ clusters are used as the simplest examples to illustrate the view of the elementary blocks introduced in GUM. The molecular orbital analysis showed that the HOMO-30 and HOMO-31 of the D 2 d Au 6 2+ core in [Au 6 (dppp) 4 ] 2+ (dppp = 1,3-Bis(diphenylphosphino)propane) [5] can be viewed as the anti-bonding and bonding orbitals of two HOMO-15 of the Au 3 + cluster (Fig. 2a ), respectively, suggesting that the HOMO-30 and HOMO-31 of the D 2 d Au 6 2+ can be viewed as the linear combination of two 1 S orbitals of Au 3 (2 e ). Similar behavior can be seen in the HOMO (Fig. 2d ) and HOMO-1 (Fig. 2e ) of the ligand-protected [Au 6 (dppp) 4 ] 2+ . Thus, we use this simple example to demonstrate that the ligand-protected [Au 6 (dppp) 4 ] 2+ and associated D 2 d Au 6 2+ core can be well described by GUM in terms of the elementary block Au 3 (2 e ). Fig. 2 The anti-bonding and bonding orbital diagrams of clusters. a D 2 d Au 6 2+ , b D 2 h Au 6 2+ , and c Mg 2 . The HOMO d and HOMO-1 e of [Au 6 (dppp) 4 ] 2+ , HOMO f , and HOMO-18 g of [Au 6 (PR 3 ) 6 ] 2+ . Color code: Au—magenta, Mg—green Full size image Likewise, the HOMO-30 and HOMO-31 of the D 2 h Au 6 2+ core of [Au 6 (PR 3 ) 6 ] 2+ [6] can be viewed as the anti-bonding and bonding orbitals of two HOMO-20 of Au 4 2+ cluster (Fig. 2b ), respectively, suggesting that the HOMO-30 and HOMO-31 of the D 2 h Au 6 2+ can be viewed as a linear combination of two 1 S orbitals of Au 4 (2 e ). Similar behavior can be seen in the HOMO (Fig. 2f ) and HOMO-18 (Fig. 2g ) of the ligand-protected [Au 6 (PR 3 ) 6 ] 2+ . Again, the ligand-protected [Au 6 (PR 3 ) 6 ] 2+ and its D 2 h Au 6 2+ core can be described by GUM as well. Finally, we note that the orbital analyses on [Au 6 (dppp) 4 ] 2+ and [Au 6 (PR 3 ) 6 ] 2+ are quite similar to that on Mg 2 , in which 3 s orbital (HOMO) of two Mg atoms can form the bonding (HOMO-1) and anti-bonding (HOMO) orbitals of Mg 2 , as shown in Fig. 2c . Summary and perspective : With introducing two groups of elementary blocks in the GUM, Au 3 (2 e ), and Au 4 (2 e ), a variety of ligand-protected gold nanoclusters, e.g., spherical and non-spherical, or magic-number and non-magic-number, can be viewed as an aggregate of the elementary groups by applying electron counting rule, a notion analog to Mingo’s united atom model for understanding weakly bound condensed icosahedra with 8 e valence electrons for each unit [7] . A recent experiment showed that the localization effect is highly important for the interpretation of the spectroscopy of gold nanoclusters [8] . Moreover, the triangle Au 3 and tetrahedral Au 4 can be considered as the basic units of face-centered cubic bulk gold. As such, one may view the ligand-protected gold clusters as the trapped intermediates on the path toward the bulk phase, but being stabilized by the ligands bounded to the surface metal atoms. A similar view has been reported previously for Al and Ga clusters [9] . In closing, GUM provides a generic, empirical, and coarse-grained model to understand and to assess the structural stabilities and structural evolution of ligand-protected gold clusters, a model that may be extended beyond gold. The reaction pathway for the Au + + Au 3 + ← → Au 4 2+ reaction in Fig. 1 was computed using DFT methods with the TPSS functional [10] and pseudopotential basis set LANL2DZ for Au, as implemented in the Gaussian 09 program package [11] . The orbitals of nanoclusters shown in Fig. 2 were computed based on the DFT method implemented in DMol 3 [12] , [13] . The generalized gradient approximation with the Perdew–Burke–Ernzerhof (PBE) [14] functional and the double numeric polarized (DNP) basis set coupled with semi-core pseudopotential were employed.